Determination ofin vivoRNA structure in low-abundance transcripts RNA structure plays important roles in diverse biological processes. However, the structures of all but the few most abundant RNAs are presently unknown in vivo . Here we introduce DMS/SHAPE-LMPCR to query the in vivo structures of low-abundance transcripts. DMS/SHAPE-LMPCR achieves attomole sensitivity, a 100,000-fold improvement over conventional methods. We probe the structure of low-abundance U12 small nuclear RNA (snRNA) in Arabidopsis thaliana and provide in vivo evidence supporting our derived phylogenetic structure. Interestingly, in contrast to mammalian U12 snRNAs, the loop of the SLIIb in U12 snRNA is variable among plant species, and DMS/SHAPE-LMPCR determines it to be unstructured. We reveal the effects of proteins on 25S rRNA, 5.8S rRNA and U12 snRNA structure, illustrating the critical importance of mapping RNA structure in vivo . Our universally applicable method opens the door to identifying and exploring the specific structure-function relationships of the multitude of low-abundance RNAs that prevail in living cells. RNA is of central importance in gene regulation, catalysis and the origin of life [1] . Numerous classes of RNA perform key biological functions via folding into diverse structures. Knowledge of RNA structure in vivo therefore provides important insights regarding the evolution and function of biological systems. For decades, chemical and enzymatic probing have been among the most common and powerful assays available to obtain structural information on RNA at nucleotide resolution [2] , [3] , [4] , [5] . This information can dramatically improve secondary structure prediction [6] , [7] , [8] . Structures generated provide insights regarding the control of RNA transcription, processing, translation and ligand-binding. Among RNA structural probing reagents, dimethyl sulfate (DMS) is highly versatile and useful for in vivo probing [9] , owing to its ability to penetrate cells and modify RNA in numerous organisms [10] , [11] , [12] , [13] , [14] , [15] , [16] . Recently, in vivo SHAPE reagents were developed and have been used to probe the highly abundant 5S rRNA in bacteria, yeast, fly and mammalian cells [17] . DMS methylates the N1 of adenine and the N3 of cytosine on the Watson–Crick base pairing face of unstructured regions such as loops, bulges and mismatches [12] , [14] , whereas SHAPE reagents acylate the 2′-hydroxyl group on the ribose sugar of unstructured regions of all four nucleotides [17] , [18] . Methylation or acylation chemistry is detected by reverse transcription (RT) stops one nucleotide before the modified nucleotide [12] , [14] , [17] , [18] , [19] . In cellular systems, structures of high-abundance RNAs such as rRNA can be assessed in vivo by a DMS/SHAPE-RT approach [11] , [12] , [14] , [17] . However, the vast majority of RNAs is of low abundance in vivo and cannot be explored by an RT-based approach. As such, very little is known about the in vivo structures of myriad RNAs, including most mRNAs and non-coding (nc) RNAs, despite their essential roles in protein synthesis and other cellular processes. Moreover, the effects of RNA-binding proteins on in vivo RNA structures are also largely unexplored. This lack of in vivo RNA structural information becomes even more evident in plants, where only a few in vivo RNA structural probing studies have been conducted, and these have been on high-abundance rRNA and photosynthesis-related RNAs [11] , [13] . In order to probe the structures of low-abundance RNAs in living cells, we developed a sensitive method that is able to detect rare RT products. This method increases the sensitivity of detection 100,000-fold over the conventional RT-based method. We demonstrate that both DMS and SHAPE chemistries permit in vivo RNA structural probing in Arabidopsis thaliana , an important model plant species and eukaryote. Notably, we employ the in vivo SHAPE reagent, 2-methylnicotinic acid imidazolide (NAI) [17] , and present the first examples of in vivo SHAPE probing in plants. We use the RT-based method ( Fig. 1 , first three steps) to successfully query the structures of rRNA (25S rRNA and 5.8S rRNA) and chloroplast mRNA ( PSBA ) in A. thaliana . We then develop a selective amplification strategy to establish a highly sensitive and robust method, ‘DMS/SHAPE-LMPCR’, that achieves a 5-log enhancement in sensitivity. Using this LMPCR-based approach ( Fig. 1 , all five steps), we uncover DMS/SHAPE modification signals from low-abundance RNAs and reveal their RNA structures for the first time in vivo . We demonstrate the immediate applicability of DMS/SHAPE-LMPCR by probing the structures of a key low-abundance mRNA ( GRP3S ) and an ncRNA (U12 small nuclear RNA (snRNA)) in A. thaliana . Comparative sequence and structural analysis uncover a secondary structure for U12 snRNA in plants. Importantly, we also reveal the effects of proteins on the RNA structures within biologically important ribonucleoparticles, including a low-abundance one, by performing comparative in vitro and in vivo DMS/SHAPE analysis on 25S rRNA, 5.8S rRNA and U12 snRNA. These studies illustrate the critical importance of mapping RNA structure in living cells. 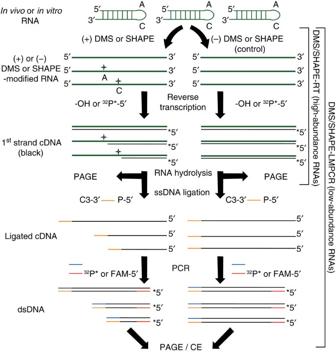Figure 1: Flowchart for targeted determination of RNA structure for high- and low-abundance RNAs. Either DMS/SHAPE-RT (Steps 1–3) or DMS/SHAPE-LMPCR can be used (all steps). In the first step, total RNA (green strand) is treated with DMS or SHAPE reagent, eitherin vitroorin vivo. In DMS/SHAPE-RT, a radiolabeled 5′-32P gene-specific primer is used for the RT step, whereas in DMS/SHAPE-LMPCR, an unlabelled 5′-OH gene-specific primer is used for the RT step. Next, the RNA is degraded by base hydrolysis. For DMS/SHAPE-LMPCR, the unlabelled cDNA (black strand) generated from RT is ligated to a DNA adaptor (orange) by single-stranded (ss) DNA ligation. Subsequently, a 5′-OH DNA adaptor-specific forward primer (blue) and a radioactive 5′-32P (for PAGE) or a 5′-FAM (for CE) gene-specific nested reverse primer (red) are used for PCR amplification of the ligated cDNA fragments. For the (−)DMS/SHAPE control reaction, all steps are the same except that DMS/SHAPE treatment is omitted. Detailed procedures for each step can be found in the Methods. Figure 1: Flowchart for targeted determination of RNA structure for high- and low-abundance RNAs. Either DMS/SHAPE-RT (Steps 1–3) or DMS/SHAPE-LMPCR can be used (all steps). In the first step, total RNA (green strand) is treated with DMS or SHAPE reagent, either in vitro or in vivo . In DMS/SHAPE-RT, a radiolabeled 5′- 32 P gene-specific primer is used for the RT step, whereas in DMS/SHAPE-LMPCR, an unlabelled 5′-OH gene-specific primer is used for the RT step. Next, the RNA is degraded by base hydrolysis. For DMS/SHAPE-LMPCR, the unlabelled cDNA (black strand) generated from RT is ligated to a DNA adaptor (orange) by single-stranded (ss) DNA ligation. Subsequently, a 5′-OH DNA adaptor-specific forward primer (blue) and a radioactive 5′- 32 P (for PAGE) or a 5′-FAM (for CE) gene-specific nested reverse primer (red) are used for PCR amplification of the ligated cDNA fragments. For the (−)DMS/SHAPE control reaction, all steps are the same except that DMS/SHAPE treatment is omitted. Detailed procedures for each step can be found in the Methods. Full size image rRNA and chloroplast mRNA structure analysis by DMS/SHAPE-RT We initially investigated rRNAs since phylogenetic structures are available for rRNA, which allows verification of the RNA structures obtained. Phylogenetic structures are derived from evolutionary relationships and provide accurate models of the in vivo , protein-associated structures of the RNA [20] , [21] . The H16–H20 region of 25S rRNA was selected for this portion of the study because its phylogenetic structure is comprised of diverse structural features including base pairs, mismatches, bulges, internal and hairpin loops and a three-helix junction ( Fig. 2 ) [22] . Our focus was to use this structurally diverse region to determine DMS and SHAPE probing in planta and to determine whether in vitro and in vivo modification patterns differ. 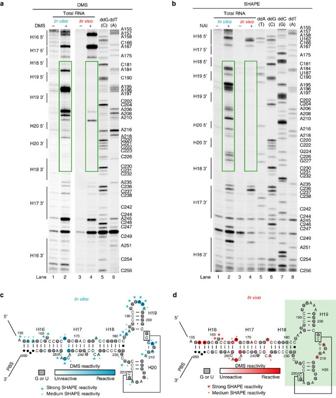Figure 2: DMS and SHAPE NAI probing of helices 16–20 of 25S rRNA reveals different modification patternsin vitroandin vivo. (a) In lanes 1–4,in vitroandin vivo,(−) or (+) DMS-RT were performed on 25S rRNA as indicated, with readout of H16–H20. Lanes 5-6 provide dideoxy sequencing. RNA input for each lane was 2 μg total RNA. (b) In lanes 1–4,in vitroandin vivo,(−) or (+) SHAPE-RT were performed on 25S rRNA as indicated, with readout of H16–H20. Lanes 5–8 provide dideoxy sequencing. RNA input for each lane was 2 μg total RNA. The green outline indicates the region ofin vivoprotein protection. (c,d) Normalizedin vitroandin vivoDMS and SHAPE reactivity mapped onto the phylogenetic structure of the H16–H20 region of 25S rRNA22. The green-shaded box indindicates the region ofin vivoprotein protection. Nucleotides replaced by black dots represent regions where confident assignment of reactivity cannot be obtained due to proximity to the primer-binding site (PBS). Figure 2: DMS and SHAPE NAI probing of helices 16–20 of 25S rRNA reveals different modification patterns in vitro and in vivo . ( a ) In lanes 1–4, in vitro and in vivo, (−) or (+) DMS-RT were performed on 25S rRNA as indicated, with readout of H16–H20. Lanes 5-6 provide dideoxy sequencing. RNA input for each lane was 2 μg total RNA. ( b ) In lanes 1–4, in vitro and in vivo, (−) or (+) SHAPE-RT were performed on 25S rRNA as indicated, with readout of H16–H20. Lanes 5–8 provide dideoxy sequencing. RNA input for each lane was 2 μg total RNA. The green outline indicates the region of in vivo protein protection. ( c , d ) Normalized in vitro and in vivo DMS and SHAPE reactivity mapped onto the phylogenetic structure of the H16–H20 region of 25S rRNA [22] . The green-shaded box in d indicates the region of in vivo protein protection. Nucleotides replaced by black dots represent regions where confident assignment of reactivity cannot be obtained due to proximity to the primer-binding site (PBS). Full size image First, we determined DMS and SHAPE modification patterns of the H16–H20 region of 25S rRNA in vitro . The in vitro DMS and SHAPE modifications occurred primarily on or near nucleotides that are single-stranded in the phylogenetic secondary structure ( Fig. 2a–c , blue). Next, we examined DMS and SHAPE modification patterns of the H16–H20 region of 25S rRNA in vivo. We first carried out a set of experiments to assure that RNA probing occurs in vivo and not during the subsequent isolation of the RNA. We began by treating intact A. thaliana seedlings with DMS or SHAPE reagent (NAI) and reading out the resultant RNA modifications using RT. For DMS, treatment for 15 min with 0.75% (~75 mM) DMS led to obvious in vivo DMS modification of 5.8S rRNA ( Supplementary Fig. S1 ). For SHAPE, NAI treatment of 15 min at 100 mM yielded ideal modification results ( Supplementary Fig. S2 ). Importantly, we found that all RNA modification occurs in vivo and not during the subsequent isolation of the RNA. This was ascertained using an exogenous RNA synthesized by in vitro T7 RNA transcription that was doped into the biological sample at the first step of total RNA extraction and then assessed for the extent of its DMS/SHAPE modification ( Supplementary Fig. S3 ). Together, these experiments confirmed that all DMS or SHAPE modification of the RNAs occurred in planta . Results of in vivo probing of the H16–H20 region of 25S rRNA are provided in Fig. 2a,b and d (red), and comparison with in vitro probing ( Fig. 2a–c ) is given as a line plot in Supplementary Fig. S4 . We found that most of the nucleotides near helices H16, H17 and H18 that were reactive in vitro were also modified in vivo ( Fig. 2 and Supplementary Fig. S4 ). Conversely, many nucleotides near H19 and H20 that were strongly modified in vitro were either not modified or modified much less strongly in vivo ( Fig. 2 and Supplementary Fig. S4 ). Low Pearson correlation coefficients (PCC) between in vitro and in vivo normalized reactivities for both DMS (PCC=0.32) and SHAPE (PCC=0.24) data indicate that RNAs have different accessibility to structural probing reagents in living cells as compared with test tube conditions ( Fig. 2 and Supplementary Fig. S4 ). We further examined the crystal structure of the ribosome, using the yeast ribosome [23] as no A. thaliana ribosome crystal structure is presently available. (Yeast ribosomal proteins are evolutionarily conserved with A. thaliana and other eukaryotes [24] ). We identified several ribosomal proteins near H18–H20 ( Fig. 2d , green shading). This observation suggests that the in vivo modification pattern observed near H19 and H20 is likely due to protein-induced protections ( Fig. 2 and Supplementary Fig. S4 , green boxes). While extensive protections were observed in this region, we also noted slightly enhanced reactivity (deprotection) on several residues—A157-A158 and C166-A167—in in vivo DMS, supporting a protein-induced RNA structural rearrangement in vivo . In summary, the primary differences between the in vitro and in vivo reactivities of the H16–H20 region of 25S rRNA stem from ribosomal protein-induced protections in vivo . We also compared 5.8S rRNA structure in vitro and in vivo, using DMS-RT in the background of total RNA ( Fig. 3a ). Extensive protections and deprotections were found in vivo as compared with in vitro . These features are readily apparent by comparing the in vitro and in vivo DMS-modified lanes in the raw data ( Fig. 3a , blue and red dots). This comparison yielded a PCC of just 0.26 ( Fig. 3b ) indicating that the structure of the RNA in vivo is very different from in vitro . Much of the weak correlation, in this instance, is likely due to the presence of intermolecular RNA–RNA interactions in the cellular environment, as part of 5.8S rRNA is known to base pair with 25S rRNA [24] (see the phylogenetic structure in Fig. 3c ). Indeed, the 5′-portion of 5.8S rRNA (H1 and H2 5′ in Fig. 3a ) was modified only in vitro , suggesting that, despite being in a background of total RNA, 5.8S rRNA is unable to base pair with 25S rRNA in vitro . To further investigate 5.8S rRNA folding in vitro , we performed DMS probing of 5.8S rRNA prepared by in vitro T7 transcription instead of by extraction from plants. The PCC between normalized DMS reactivities of in vitro 5.8S rRNA from T7 transcription versus in vitro 5.8S rRNA from total RNA was very strong (PCC=0.87), while the correlation between in vitro 5.8S rRNA from the T7 transcription and in vivo 5.8S rRNA was exceptionally weak (PCC=0.14) ( Fig. 3b ). These results further support the conclusion that 5.8S rRNA folds very differently in vitro and in vivo and that ribosomal proteins are important cellular factors required for the stabilization of 25 rRNA–5.8S rRNA interactions [25] . 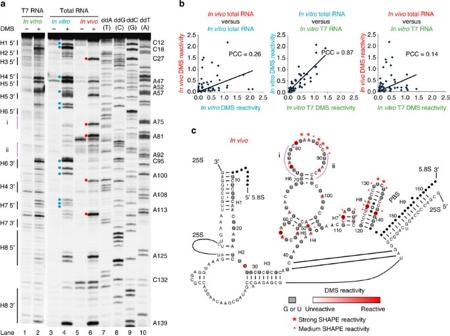Figure 3: DMS probing of 5.8S rRNA yields different RNA structuresin vitroandin vivo. (a) In lanes 1–6, DMS-RT was performed onin vitro5.8S rRNA from T7 transcription (T7 RNA),in vitrototal RNA, orin vivototal RNA, in each case using a 5.8S rRNA-gene-specific primer. Lanes 7–10 provide dideoxy sequencing. Blue and red dots denote key nucleotides ofin vitro-only (i.e., protectedin vivo) andin vivo-only (i.e., deprotectedin vivo) DMS modifications. (b) Correlation plots of 5.8S rRNA fromin vivototal RNA versusin vitrototal RNA, 5.8S rRNA fromin vitrototal RNA versusin vitroT7 transcription and 5.8S rRNA fromin vivototal RNA versusin vitroT7 transcription. PCC are provided on each plot. (c) Normalizedin vivoDMS and SHAPE probing results mapped onto the phylogenetic structure of 5.8S rRNA22. Two proposed regions (i and ii) of ribosomal protein protection (a,c, purple) are supported by bothin vivoDMS andin vivoSHAPE probing results (SeeaandSupplementary Fig. S2). Nucleotides replaced by black dots represent regions where confident assignment of reactivity cannot be obtained due to proximity to the PBS or 5′ end of the 5.8 s rRNA. Certain nucleotides in 25S rRNA that do not interact with 5.8S rRNA are represented by a black curve. Figure 3: DMS probing of 5.8S rRNA yields different RNA structures in vitro and in vivo . ( a ) In lanes 1–6, DMS-RT was performed on in vitro 5.8S rRNA from T7 transcription (T7 RNA), in vitro total RNA, or in vivo total RNA, in each case using a 5.8S rRNA-gene-specific primer. Lanes 7–10 provide dideoxy sequencing. Blue and red dots denote key nucleotides of in vitro -only (i.e., protected in vivo ) and in vivo -only (i.e., deprotected in vivo ) DMS modifications. ( b ) Correlation plots of 5.8S rRNA from in vivo total RNA versus in vitro total RNA, 5.8S rRNA from in vitro total RNA versus in vitro T7 transcription and 5.8S rRNA from in vivo total RNA versus in vitro T7 transcription. PCC are provided on each plot. ( c ) Normalized in vivo DMS and SHAPE probing results mapped onto the phylogenetic structure of 5.8S rRNA [22] . Two proposed regions (i and ii) of ribosomal protein protection ( a , c , purple) are supported by both in vivo DMS and in vivo SHAPE probing results (See a and Supplementary Fig. S2 ). Nucleotides replaced by black dots represent regions where confident assignment of reactivity cannot be obtained due to proximity to the PBS or 5′ end of the 5.8 s rRNA. Certain nucleotides in 25S rRNA that do not interact with 5.8S rRNA are represented by a black curve. Full size image Our in vivo DMS-RT data on 5.8S rRNA are consistent with the phylogenetic structure. We also observed that some single-stranded regions in the 5.8S rRNA phylogenetic structure had low DMS reactivity, suggesting that these regions are protected by cellular factors in vivo ( Fig. 3c ). To investigate this possibility, we further performed in vivo modification on 5.8S rRNA with SHAPE and found that these single-stranded regions have low SHAPE reactivities, consistent with our DMS findings ( Supplementary Fig. S2 ). Next, we examined the crystal structure of the yeast ribosome [23] and identified several ribosomal proteins adjacent to 5.8S rRNA, suggesting that the low DMS and SHAPE reactivities in those regions in A. thaliana are caused by protein-induced protections. Two such single-stranded regions, ‘i’ and ‘ii’ in Fig. 3c , have been reported as protected from DMS modification in yeast but deprotected in the absence of yeast ribosomal protein L26 (ref. 26 ), supporting the hypothesis that those single-stranded regions in 5.8S rRNA with low DMS/SHAPE reactivities are protected by ribosomal proteins. In sum, our results illustrate that DMS and SHAPE can target and report native 5.8S rRNA secondary structure in living cells and that this structure is markedly different from in vitro structures. We next sought to test whether in vivo SHAPE can target important chloroplast mRNA of unknown structure. We chose the 5′UTR of PSBA (Atcg00020.1), a vital chloroplast mRNA that encodes the D1 protein of the photosystem II reaction center. We first performed DMS-RT ( Fig. 4a ), as DMS has previously been shown to target chloroplast mRNA in a green alga [13] . We constructed the secondary structure of the 5′UTR of PSBA from A. thaliana using normalized DMS reactivities as constraints ( Fig. 4b and see Methods ). It has been reported that the highly conserved AU box in the 5′UTR of PSBA is crucial in translation, as mutation or deletion of this region leads to a drastic decrease in translation yield [27] . We found that the A nucleotides in this box are highly reactive to DMS in vivo , indicating that the nucleotides in this loop are unstructured ( Fig. 4 ). We then performed in vivo SHAPE-RT and obtained modifications that support the DMS-constrained structure ( Fig. 4 ), demonstrating that NAI can target chloroplast mRNAs. Combining our in vivo finding on the unstructured AU box with the mutational study [27] , it appears that the AU box in the 5′UTR of PSBA may be a regulatory site in vivo , e.g., for protein binding in a redox-dependent fashion as is known to occur at the 5′ UTR of PSBA [28] . In sum, we demonstrated that SHAPE can modify chloroplast mRNA in vivo and identified important structural features that agree with in vivo DMS probing. 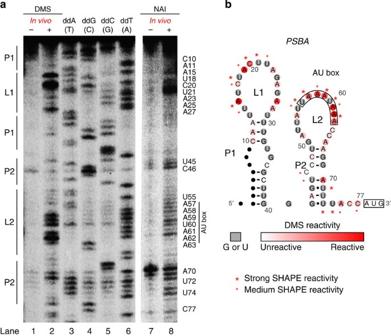Figure 4: DMS/SHAPE-RT probing and 5′UTR secondary structure ofPSBA. (a)In vivoDMS (lanes 1–2) and SHAPE (lanes 7–8) probing of the complete 5′UTR ofPSBAvia DMS/SHAPE-RT. Lanes 3–6 show dideoxy sequencing. Owing to its lower abundance in cells in comparison with 5.8S rRNA (Fig. 5b), a minimum of 15 μg of total RNA was needed for each lane to allow the detection of DMS/SHAPE modifications ofPSBA5′UTR via the DMS/SHAPE-RT assay. (b) Normalizedin vivoDMS-constrained secondary structures of 5′UTR ofPSBA(seeMethods). The AU box is enclosed with a black outline. The SHAPE reactivity was overlaid onto the secondary structure and is highly consistent with the structure, indicating thatin vivoSHAPE reagent (NAI) can target chloroplast mRNAs in plant systems. Nucleotides replaced with black dots represent regions where confident assignment of reactivity cannot be obtained due to proximity to the 5′ end of the RNA. Figure 4: DMS/SHAPE-RT probing and 5′UTR secondary structure of PSBA . ( a ) In vivo DMS (lanes 1–2) and SHAPE (lanes 7–8) probing of the complete 5′UTR of PSBA via DMS/SHAPE-RT. Lanes 3–6 show dideoxy sequencing. Owing to its lower abundance in cells in comparison with 5.8S rRNA ( Fig. 5b ), a minimum of 15 μg of total RNA was needed for each lane to allow the detection of DMS/SHAPE modifications of PSBA 5′UTR via the DMS/SHAPE-RT assay. ( b ) Normalized in vivo DMS-constrained secondary structures of 5′UTR of PSBA (see Methods ). The AU box is enclosed with a black outline. The SHAPE reactivity was overlaid onto the secondary structure and is highly consistent with the structure, indicating that in vivo SHAPE reagent (NAI) can target chloroplast mRNAs in plant systems. Nucleotides replaced with black dots represent regions where confident assignment of reactivity cannot be obtained due to proximity to the 5′ end of the RNA. Full size image Development of attomole sensitivity LMPCR-based assay The RNA structures described above were assayed via an RT-based approach. However, this approach suffers from being insensitive. It can detect only the relatively few high-abundance transcripts, such as rRNAs and PSBA ( Figs 2 , 3 , 4 ), which make up only a very small fraction of all the distinct transcripts in cells. As such, it is important to develop a more sensitive method to determine RNA structure of low-abundance transcripts in vivo . We first determined the sensitivity limits of the standard in vivo RT-based assay, using DMS probing reagent as an example. The total input RNA was serially diluted until the observable DMS modification pattern for 5.8S rRNA was lost. We found that a relatively large amount of 5.8S rRNA (~1 pmol) is necessary for conventional DMS-RT ( Fig. 5a ). This is approximately the amount of 5.8S rRNA found in 2 μg of a ‘total RNA’ extraction, which immediately presents a problem if one wants to assay the many much lower abundance RNAs. Without a new approach an RNA at 100,000-fold lower abundance than 5.8S rRNA would require ~0.2 g of total RNA input for the DMS-RT assay, which is clearly impractical. To improve sensitivity, we explored and developed an amplification-based method, which we refer to as ‘DMS/SHAPE-LMPCR’ ( Fig. 1 , all steps). In this approach, a DNA adaptor is ligated to the 3′ end of the complementary DNA (cDNA), and the ligated cDNA is PCR amplified using a gene-specific and an adaptor-specific primer. With this approach, we found that the DMS modification pattern of 5.8S rRNA is observable even at a 10-attomole (10 −17 ) level of 5.8S rRNA input ( Fig. 5a ), which represents a remarkable 100,000-fold enhancement in sensitivity. Notably, the modification pattern derived from DMS-LMPCR was consistent with the pattern derived from the standard DMS-RT data ( Fig. 5a , compare lane 3 with 5 and 7), with strong PCC between the normalized DMS reactivities for different regions of 5.8S rRNA ranging from 0.72 to 0.82. 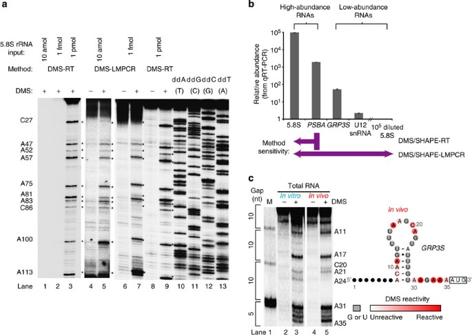Figure 5: Development and application of attomole sensitivity LMPCR-based assay. (a) Enhanced sensitivity of DMS-LMPCR allows detection of DMS modification of attomole quantities of RNA. Two micrograms total RNA (equal to ~1 pmol of 5.8S rRNA, lane 3) ofin vivoDMS-treated total RNA was serially diluted to amounts containing an estimated 1 fmol (lane 2) or 10 amol (lane 1) of 5.8S rRNA and used for reverse transcription. The sensitivity of DMS-RT was determined to be ~1 pmol of the target RNA. A similar test was performed to determine DMS-LMPCR sensitivity. Two μg total RNA ofin vivo(−)DMS- or (+)DMS-treated total RNA was serially diluted to amounts containing an estimated 1 pmol (lanes 8–9), 1 fmol (lanes 6–7) or 10 amol (lanes 4–5) of 5.8S rRNA, and then DMS-LMPCR was performed on 5.8S rRNA. The sensitivity of DMS-LMPCR was determined to be ~10 amol. Lanes 10–13 provide dideoxy sequencing. The asterisks were used for tracking of the bands from different lanes. (b) qRT-PCR analysis of relative abundance of selected RNA candidates. 5.8S rRNA was used as a reference. Error bars represent the s.d. of three biological replicates. Ranges of sensitivity of the DMS/SHAPE-RT and DMS/SHAPE-LMPCR approaches are shown beneath the graph. Low-abundance RNA was defined as inability to detect by DMS/SHAPE-RT. (c) DMS-LMPCR reveals structural aspects of a low-abundance RNA transcript. Lanes 2–5 showin vitroandin vivoDMS probing of the completeGRP3S5′UTR via DMS-LMPCR. A 10 nt marker (M) was size fractionated (lane 1) to allow nucleotide assignment based on spacing. RNA input for DMS-LMPCR was 1 μg of total RNA.In vitroandin vivoDMS modifications were similar (compare lanes 3 and 5),with a PCC of 0.84 betweenin vitroandin vivoDMS reactivities.In vivoDMS-constrained secondary structure ofGRP3S5′UTR is shown at right. (In vitroDMS-constrained structure was identical.) Nucleotides replaced by black dots represent regions where confident assignment of reactivity cannot be obtained due to proximity to the 5′ end of the RNA. Figure 5: Development and application of attomole sensitivity LMPCR-based assay. ( a ) Enhanced sensitivity of DMS-LMPCR allows detection of DMS modification of attomole quantities of RNA. Two micrograms total RNA (equal to ~1 pmol of 5.8S rRNA, lane 3) of in vivo DMS-treated total RNA was serially diluted to amounts containing an estimated 1 fmol (lane 2) or 10 amol (lane 1) of 5.8S rRNA and used for reverse transcription. The sensitivity of DMS-RT was determined to be ~1 pmol of the target RNA. A similar test was performed to determine DMS-LMPCR sensitivity. Two μg total RNA of in vivo (−)DMS- or (+)DMS-treated total RNA was serially diluted to amounts containing an estimated 1 pmol (lanes 8–9), 1 fmol (lanes 6–7) or 10 amol (lanes 4–5) of 5.8S rRNA, and then DMS-LMPCR was performed on 5.8S rRNA. The sensitivity of DMS-LMPCR was determined to be ~10 amol. Lanes 10–13 provide dideoxy sequencing. The asterisks were used for tracking of the bands from different lanes. ( b ) qRT-PCR analysis of relative abundance of selected RNA candidates. 5.8S rRNA was used as a reference. Error bars represent the s.d. of three biological replicates. Ranges of sensitivity of the DMS/SHAPE-RT and DMS/SHAPE-LMPCR approaches are shown beneath the graph. Low-abundance RNA was defined as inability to detect by DMS/SHAPE-RT. ( c ) DMS-LMPCR reveals structural aspects of a low-abundance RNA transcript. Lanes 2–5 show in vitro and in vivo DMS probing of the complete GRP3S 5′UTR via DMS-LMPCR. A 10 nt marker (M) was size fractionated (lane 1) to allow nucleotide assignment based on spacing. RNA input for DMS-LMPCR was 1 μg of total RNA. In vitro and in vivo DMS modifications were similar (compare lanes 3 and 5),with a PCC of 0.84 between in vitro and in vivo DMS reactivities. In vivo DMS-constrained secondary structure of GRP3S 5′UTR is shown at right. ( In vitro DMS-constrained structure was identical.) Nucleotides replaced by black dots represent regions where confident assignment of reactivity cannot be obtained due to proximity to the 5′ end of the RNA. Full size image mRNA and ncRNA structural analysis by DMS/SHAPE-LMPCR We sought to determine whether DMS-LMPCR can reveal DMS modifications of low-abundance transcripts that cannot be detected and analysed by conventional DMS-RT. We interrogated a low-abundance RNA, GRP3S (At2g05380.1), which encodes the short isoform of glycine-rich protein 3. Glycine-rich protein 3 short isoform (GRP3S) interacts with a plant cell wall-associated kinase, suggesting a role in signal transduction; other glycine-rich proteins have been implicated in plant defence and response to abiotic stress [29] . The level of GRP3S is ~1,900-fold lower than that of 5.8S rRNA according to quantitative reverse transcriptase PCR (qRT-PCR) ( Fig. 5b ). We used 1 μg of total RNA for each reaction and performed in vitro and in vivo DMS-LMPCR probing on the complete 35 nt 5′UTR of GRP3S . As shown in Fig. 5c , DMS modifications on this low-abundance RNA transcript were obtained. The in vitro and in vivo DMS modification patterns were similar ( Fig. 5c , compare lanes 3 and 5), with a strong PCC=0.84 between normalized DMS reactivity under the two conditions. Despite the similarities, minor differences occur. These are found at nucleotides C20 and A24, with C20 being more reactive in vivo , and A24 being somewhat less reactive in vivo . Both in vitro and in vivo DMS-constrained structure determination yielded the same secondary structure, consisting of a hairpin with 6 bp in the stem and 10 nt in the loop ( Fig. 5c ). Inspecting the structure suggests that the minor differences in modification patterns may arise from loop dynamics and breathing of the closing base pair in vitro . Finally, we studied an RNA whose abundance approaches our benchmark sensitivity ( Fig. 5b ), using both DMS and SHAPE probing reagents. We interrogated U12 snRNA (At1g61275.1), which is a nc snRNA of the minor spliceosomal complex [30] , responsible for the splicing of a divergent class of pre-mRNA introns. The level of U12 snRNA in A. thaliana is ~45,000-fold lower than that of 5.8S rRNA according to qRT-PCR ( Fig. 5b ). We also conducted a comparative sequence analysis of U12 snRNAs across vascular plant and moss genomes, which revealed that U12 snRNA sequences are highly conserved ( Fig. 6a , top). We found that covariation in multiple base pairs exists across these species ( Fig. 6a , top), providing evidence for conserved structural domains in U12 snRNA. On the basis of these sequences, we derived a phylogenetic structure of plant U12 snRNA ( Fig. 6b ). The resultant plant U12 snRNA structures are similar to mammalian U12 snRNA structures [31] ( Fig. 6a , bottom and Fig. 6c ), providing evolutionary support for our proposed U12 phylogenetic structure in plants ( Fig. 6b ). Our plant U12 snRNA phylogenetic structure shows that SLIII elements form a single and long hairpin at the 3′end, consistent with human U12 snRNA [31] ( Fig. 6b,c ). 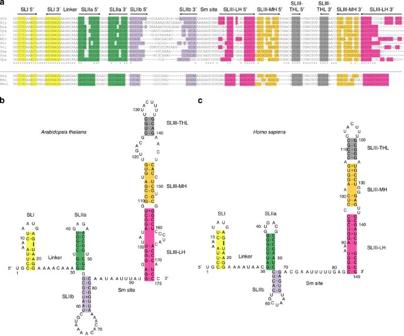Figure 6: Comparative sequence analysis of plant and mammalian U12 snRNA reveals conserved secondary structure. (a) Comparative sequence analysis on 11 U12 snRNAs from plant species with well-sequenced genomes (top) yields conserved secondary structural domains. (Ath:Arabidopsis thaliana; Aly:Arabidopsis lyrata;Bra:Brassica rapa;Cpa:Carica papaya;Ccl:Citrus clementina;Mtr:Medicago truncatula;Ptr:Populus trichocarpa;Vvi:Vitis vinifera;Zma:Zea mays;Osa:Oryza sativa;Ppa:Physcomitrella patens)Three mammalian U12 snRNAs (bottom) are shown for comparison. (Hsa:Homo sapiens;Mmu:Mus musculus;Mmul:Macaca mulatta). Asterisks denote conserved nucleotides. (b,c) Similar RNA phylogenetic structures ofA. thalianaandHomo sapiensU12 snRNA. (b) Phylogenetic structure of plant U12 snRNA inA. thaliana, constructed based on the sequences of the 11 plant U12 snRNAs shown ina(top). (c) Phylogenetic structure of mammalian U12 snRNA, as reported previously31. The stems are coloured according toato allow easier comparison betweenA. thalianaandH. sapiensU12 snRNA. This structure is also supported by comparison of the three mammalian U12 snRNAs (a, bottom). (SeeSupplementary Table 1for gene information). Figure 6: Comparative sequence analysis of plant and mammalian U12 snRNA reveals conserved secondary structure. ( a ) Comparative sequence analysis on 11 U12 snRNAs from plant species with well-sequenced genomes (top) yields conserved secondary structural domains. (Ath: Arabidopsis thaliana ; Aly: Arabidopsis lyrata; Bra: Brassica rapa; Cpa: Carica papaya; Ccl: Citrus clementina; Mtr: Medicago truncatula; Ptr: Populus trichocarpa; Vvi: Vitis vinifera; Zma: Zea mays; Osa: Oryza sativa; Ppa: Physcomitrella patens) Three mammalian U12 snRNAs (bottom) are shown for comparison. (Hsa: Homo sapiens; Mmu: Mus musculus; Mmul: Macaca mulatta ). Asterisks denote conserved nucleotides. ( b , c ) Similar RNA phylogenetic structures of A. thaliana and Homo sapiens U12 snRNA. ( b ) Phylogenetic structure of plant U12 snRNA in A. thaliana , constructed based on the sequences of the 11 plant U12 snRNAs shown in a (top). ( c ) Phylogenetic structure of mammalian U12 snRNA, as reported previously [31] . The stems are coloured according to a to allow easier comparison between A. thaliana and H. sapiens U12 snRNA. This structure is also supported by comparison of the three mammalian U12 snRNAs ( a , bottom). (See Supplementary Table 1 for gene information). Full size image Both DMS and SHAPE target the predicted single-stranded regions of A. thaliana U12 snRNA ( Fig. 7a,b and Supplementary Fig. S5 ), supporting our derived structural model ( Fig. 7c,d ). U12 snRNA interacts with Sm proteins to form the small nuclear ribonucleoparticle. A striking protection pattern occurs at the Sm protein-binding site uniquely in vivo , which is most visible in the SHAPE probing ( Fig. 7b,d and Supplementary Fig. S5b , green box). The Sm site has a conserved sequence of RAU 4-6 GR [32] , [33] , and 2′-hydroxyl groups and uridine bases have been reported to be especially important for stable small nuclear ribonucleoparticle formation [32] . Uridine is probed uniquely by SHAPE as are the 2′-hydroxyl groups, showing that DMS and SHAPE are complementary reagents in vivo . These results reveal specific protein-binding sites on a low-abundance ncRNA in vivo . 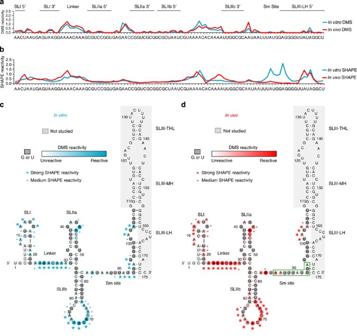Figure 7: DMS/SHAPE-LMPCR uncoversin vivostructural aspects of minor spliceosomal U12 snRNA. (a,b) DMS and SHAPE reactivity plots of U12 snRNA using data fromSupplementary Fig. S5. Different regions of the U12 snRNA are annotated above the plot in (a). (c,d)In vitroandin vivoDMS/SHAPE reactivity mapped onto the phylogenetic structure of plant U12 snRNA. The proposed Sm protein-binding site is indicated by a green outline. RNA regions that are used for the two primer-binding sites and that are close to the 5′- and 3′-ends cannot be assessed; these regions are shaded with a light-grey box. Figure 7: DMS/SHAPE-LMPCR uncovers in vivo structural aspects of minor spliceosomal U12 snRNA. ( a , b ) DMS and SHAPE reactivity plots of U12 snRNA using data from Supplementary Fig. S5 . Different regions of the U12 snRNA are annotated above the plot in ( a ). ( c , d ) In vitro and in vivo DMS/SHAPE reactivity mapped onto the phylogenetic structure of plant U12 snRNA. The proposed Sm protein-binding site is indicated by a green outline. RNA regions that are used for the two primer-binding sites and that are close to the 5′- and 3′-ends cannot be assessed; these regions are shaded with a light-grey box. Full size image Finally, to demonstrate the capability of our method for higher throughput, we coupled it with capillary electrophoresis (CE) by performing DMS-LMPCR on U12 snRNA using a fluorescent primer ( Supplementary Fig. S6 ). The CE data strongly correlate with the polyacrylamide gel electrophoresis (PAGE) data, with a PCC of 0.76 between these two methods. This opens the door to higher throughput of the method, as established for in vitro SHAPE experiments [34] , [35] . In sum, our establishment of the ultrasensitive DMS/SHAPE-LMPCR method allows interrogation of the structures of rare biological transcripts, which is not possible by prior RT-based methods. There are three key technical advantages of DMS/SHAPE-LMPCR. First, it requires only simple RNA sample handling and preparation; thus, costly and time-consuming steps of selective enrichment of the RNA of interest or, conversely, depletion of high-abundance RNAs (i.e., rRNAs) are not needed. Second, coupling between in vivo DMS/SHAPE probing and LMPCR permits critical gains in sensitivity and selectivity. In comparison with grams of total RNA required for conventional methods, 1 μg of total RNA is sufficient for this assay to probe structure of low-abundance RNA, which is readily obtained from 20 mg (fresh weight) of seedlings in our study, and a comparable amount of RNA could be obtained from routine preparation of cells or tissues of other organisms. This makes structural probing of low-abundance transcripts practical. This reduced quantitative requirement also makes it feasible to harvest the requisite amount of RNA for in vivo structure profiling on RNAs of interest in rare cell or tissue types. Third, comparison of in vivo probing results with in vitro structures, made feasible by DMS/SHAPE-LMPCR, allows the identification of nucleotides that are critical in modulating RNA structure in living cells as inferred from both differential protections and deprotections. We have explored the structures of a number of plant RNAs with differential abundance in living cells. In particular, the evolutionary and structural aspects of U12 snRNA have been elucidated, expanding our current understanding of structure of the minor spliceosomal complex in plants. Recently, a detailed RNA mutagenesis study on human U12 snRNA was performed to identify the importance of several structural elements [31] . In that study, the loop sequence of SLIIb was reported to be evolutionarily conserved, yet mutation and deletion analysis showed it to be dispensable for splicing. While we also find strong sequence conservation in this region for three mammalian U12 snRNAs ( Fig. 6a , bottom), the loop sequence and loop length of SLIIb are highly variable in plants ( Fig. 6a , top), supporting its dispensable nature in splicing [31] . Indeed, our DMS/SHAPE-LMPCR probing result showed that this loop is highly unstructured in A. thaliana U12 snRNA ( Fig. 7 ). Overall, our DMS/SHAPE-LMPCR probing on this rare ncRNA supports our proposed phylogenetic structure of U12 snRNA in plants. Another important observation on U12 snRNA is the strong protection observed in our in vivo SHAPE-LMPCR analysis, suggesting Sm protein binding to a single-stranded Sm-site in vivo . This result highlights the value of our method’s capability to probe RNA structure of rare transcripts both in vitro and in vivo, and detect important features that are uniquely present in vivo . Undoubtedly, in vitro RNA structural probing experiments using T7 transcripts or extracted total RNA are important in understanding RNA structure, and some RNAs, e.g., those lacking intermolecular interactions with proteins or other RNAs, or harbouring insensitivity to cellular ionic and crowding conditions, may exhibit the same structures in vivo and in vitro . Caution is needed, however, when in vitro and in vivo modification patterns differ. The modification patterns of 25S rRNA, 5.8S rRNAs and U12 snRNA, as demonstrated here, exemplify this phenomenon. In the case of 25S rRNA, major differences were likely due to protein-induced protection in vivo ( Fig. 2 ), while for 5.8S rRNA, folding in vitro occurred in the absence of the known base pairing with 25S rRNA [22] ( Fig. 3 ). In the case of U12 snRNA, the Sm site element was protected in vivo ( Fig. 7 ). Since in vivo and in vitro probing are complementary methods and both can identify structural features and impacts of various cellular factors on the RNA of interest, it is thus useful to perform both in vivo and in vitro probing. In this study, we have presented the first in vivo structures of several plant RNAs, having probed rRNA, chloroplast mRNA, cytosolic mRNA and nuclear ncRNA in living cells. Our sensitive and robust method allows the structural exploration of many vital categories of RNAs that have not previously been amenable to study in living cells due to limitations in sensitivity and/or RNA availability. Moreover, in vitro and in vivo comparative analysis of RNA, as facilitated by our method, reveals the effects of proteins on the RNA structures within biologically important ribonucleoparticles and offers significant biological insights into RNA structure in living cells. In summary, application of DMS/SHAPE-LMPCR has advanced current understanding of RNA structure in plants, and provides a general platform for the study of the structures of low-abundance transcripts in any organism. Preparation of in vitro T7 RNA transcripts Two in vitro T7 RNA transcripts were prepared for DMS and SHAPE control tests: 5.8S rRNA (166 nt) and a dope-in RNA (168 nt). The dope-in RNA’s primer-binding site has no significant complementarity to any RNA in A. thaliana and therefore can act as an exogeneous RNA for the DMS/SHAPE control reaction. Transcripts were produced from double-stranded DNA templates using T7 RNA polymerase. The double-stranded DNA templates were prepared from single-stranded synthetic DNA oligonucleotides (IDT, Coralville, IA) that were PCR amplified using gene-specific primers. Two Gs were appended after the T7 promoter sequence of the DNA template (at the 5′ ends of these RNAs) to improve in vitro T7 RNA transcription yields [36] . The resulting dsDNA products were fractionated on a 1.5% agarose gel for 1 h at 100 W, visualized under brief UV shadowing and purified using an E.Z.N.A. gel extraction kit (Omega Bio-Tek) following the manufacturer’s protocol. T7 RNA transcription was performed using the MEGAscript T7 Kit (Ambion) following the manufacturer’s protocol. The resulting RNA product was size fractionated on an 8.3 M urea-10% polyacrylamide gel and visualized under brief UV shadowing. The gel slice was crushed and soaked overnight at 4 °C in 10 mM Tris (pH 7.5), 1 mM EDTA and 250 mM NaCl (1X TEN 250 ) with constant rotary shaking. The gel mixture was filtered through a 0.25 μm filter and ethanol precipitated. The pellet was washed with ice-cold 70% ethanol, dissolved in RNase-free water and quantified with UV-spectroscopy. RNA was stored at −20 °C. In vitro total RNA preparation A. thaliana seeds were obtained from the Arabidopsis Biological Resource Center (ABRC, http://www.arabidopsis.org/abrc/ ) for the Columbia (Col-0) accession. Sterilization of the seeds was performed by treating with 70% (v/v) ethanol. Seeds were then plated on half-strength Murashige and Skoog (MS) medium. The seeds were stratified by storing for at 4 °C for 3 to 4 days. Subsequently, the plates were covered with aluminium foil to keep out light and kept for 5 days in a growth chamber maintained at 22–24 °C. The resulting 5-day-old A. thaliana etiolated (grown in darkness) seedlings were frozen with liquid N 2 and ground into powder using a chilled mortar and pestle precleaned with RNase Zap (Ambion). The powder was then subjected to total RNA extraction, following the protocol described in the RNeasy Plant Mini Kit (Qiagen). The extracted total RNA was then treated with TURBO DNase (Ambion) following the manufacturer’s protocol, followed by phenol chloroform extraction and ethanol precipitation. The RNA was resuspended in RNase-free water and quantified with UV-spectroscopy. In addition, the quality of the RNA was confirmed by gel electrophoresis to ensure that rRNA bands were intact. RNA was stored at −20 °C. In vitro DMS chemical probing on targeted RNA candidates All manipulations involving DMS were conducted in a chemical fume hood. In vitro T7 transcript or total extracted ( in vitro) seedling RNA was denatured at 95 °C for 1.5 min then cooled to 4 °C for 1.5 min for renaturation. An equal volume of 2X DMS reaction buffer was added to 2 pmol of T7 transcript or 1–15 μg (depending on the abundance of the RNA candidate being targeted) of total ( in vitro) seedling RNA, resulting in final 1X DMS reaction buffer concentrations of 100 mM KCl, 40 mM HEPES (pH 7.5) and 0.5 mM MgCl 2 , approximately mimicking cellular ionic conditions. The final total volume was 20 μl. The reaction was mixed thoroughly and kept at room temperature for 15 min to allow system equilibration. DMS (99.8% purity) stock (Sigma-Aldrich) was diluted (1:10 v/v) in 95% ethanol, immediately added to the reaction mixture to a final concentration of 1% (~100 mM DMS) and allowed to react with the RNA for 3 min at room temperature. RNA under this condition achieves single-hit kinetics conditions ( Fig. 3 ). To quench the reaction, freshly prepared dithiothreitol (DTT) was added to a final concentration of 0.5 M and mixed thoroughly. The reaction was immediately applied to a Micro Bio-Spin P-6 gel column (Bio-Rad) following the manufacturer’s protocol to remove small molecules, and the filtrate was subjected to ethanol precipitation. Minus DMS treatment was performed by adding 95% ethanol instead of DMS. For a quench control, DTT at a final concentration of 0.5 M was added before DMS, while the other procedures remained the same as described above (see Supplementary Information ). In vivo DMS chemical probing on targeted RNA candidates A. thaliana etiolated seedlings were grown for 5 days in the dark (see above). Seedlings were harvested with forceps and then put into 20 ml 1x DMS reaction buffer (100 mM KCl, 40 mM HEPES (pH 7.5) and 0.5 mM MgCl 2 in a 50 ml Falcon tube. Next, DMS (Sigma-Aldrich, 99.8% purity) was added to give a final concentration of 0.75% (~75 mM). The reaction proceeded for 15 min at room temperature and the seedlings were swirled periodically. Freshly prepared DTT was added to a final concentration of 0.5 M to quench the reaction. After swirling for 2 min the liquid was decanted and ~100 ml of deionized water was used to wash the seedlings. The seedlings were then frozen with liquid N 2 and ground to a powder using a mortar and pestle that had been treated with RNase Zap (Ambion). Total RNA was extracted with the RNeasy Plant Mini Kit (Qiagen). Minus DMS treatment was performed by adding deionized water instead of DMS. Two quench controls were conducted. For the first quench control, DTT at a final concentration of 0.5 M was added before DMS; the other procedures remained the same as described above. A second quench control was performed to ensure that the DTT quenching of DMS was efficient and no ‘in vitro’ DMS modification occurred during the RNA extraction process in in vivo experiments. In this control, 2 pmol of a doped-in RNA (168 nt) was added when the lysis buffer was added to the ground powder (first step of total RNA extraction); this allowed monitoring as to whether the doped-in RNA was methylated by DMS during the extraction process—a result which, had it occurred, would have led to spurious conclusions regarding the in vivo nature of the RNA structure. All extracted RNA samples were then treated with TURBO DNase (Ambion) following the manufacturer’s protocol, followed by phenol chloroform extraction and ethanol precipitation (see Supplementary Information ). Synthesis of NAI The synthesis of the SHAPE reagent NAI was performed according to the literature [17] . All manipulations involving synthesis and use of NAI were conducted in a chemical fume hood and with reagents from Sigma-Aldrich. To prepare NAI, 137 mg (1 mmol) of 2-methylnicotinic acid, alternative name 2-methylpyridine-3-carboxylic acid, was first dissolved in 500 μl anhydrous dimethyl sulfoxide (DMSO) in a 1.7 ml Eppendorf tube with brief vortexing at room temperature. In another 1.7 ml Eppendorf tube, 162 mg (1 mmol) 1,1′-carbonyldiimidazole was dissolved in 500 μl anhydrous DMSO, and this solution was added slowly to the 2-methylnicotinic acid solution over 5 min with brief vortexing. The resulting solution was vortexed briefly at room temperature with occasional opening of the cap until gas evolution was complete. The resulting solution was used as a 1.0 M stock solution containing a 1:1 mixture of SHAPE reagent NAI, and imidazole as a byproduct, without further purification according to an earlier study [17] . The solution was aliquoted and was kept frozen at −80 °C when not in use. The stock solution was thawed to room temperature before opening and use. In vitro SHAPE chemical probing on targeted RNA candidates All manipulations involving NAI were conducted in a chemical fume hood. All the procedures for in vitro SHAPE chemical probing were identical to those for in vitro DMS chemical probing described above, except that the final concentration of NAI was 50 mM and the reaction was allowed to occur for 15 min. Minus SHAPE treatment was performed by adding anhydrous DMSO instead of NAI. In vivo SHAPE chemical probing on targeted RNA candidates All the procedures for in vivo SHAPE chemical probing were identical to those for in vivo DMS chemical probing described above, except that the final concentration of NAI was 100 mM. Minus SHAPE treatment was performed by adding anhydrous DMSO instead of NAI. Gene-specific reverse transcription One pmol of in vitro T7 transcribed RNA, 1–15 μg of in vitro total RNA (the actual amount depended on the abundance of the RNA candidate being targeted) or 1–15 μg of in vivo total RNA (the actual amount depended on the abundance of the RNA candidate being targeted) was resuspended in 5.5 μl RNase-free water and mixed with either 1 μl of 2.5 μM (unlabelled) or ~200,000 counts per minute (c.p.m.) per μl of 32 P-radiolabelled DNA gene-specific primer. The solution was heated at 75 °C for 3 min, then 3 μl of reverse transcription reaction buffer was added to the mixture to a final concentration of 20 mM Tris (pH 8.3), 1 mM DTT, 8 mM MgCl 2 and 1 mM dNTPs, and the reaction was incubated at 35 °C for annealing. The reaction was then heated to 55 °C for 1 min, 0.5 μl of Superscript III reverse transcriptase (100 U total) was added, and reverse transcription was allowed to proceed for 15 min at 55 °C. Next, 1 μl of 2 M NaOH was added to the 10 μl mixture, which was heated at 95 °C for 10 min to hydrolyze all RNAs and denature reverse transcriptase. For DMS/SHAPE-RT experiments, the reverse transcription reaction mixture was mixed with an equal volume of 2X stop solution, which contained 100% deionized formamide, 20 mM Tris, pH 7.5, 40 mM EDTA as well as xylene cyanol and bromophenol blue dye for tracking. For DMS/SHAPE-LMPCR experiments, the reverse transcription reaction mixture was phenol chloroform extracted and applied to an illustra MicroSpin S-200 HR column (GE Healthcare Life Sciences) following the manufacturer’s protocol, and the cDNA in the filtrate was subjected to ethanol precipitation. Single-stranded DNA ligation The single-stranded DNA ligation condition was modified from literature [37] and manufacturer’s (Epicentre) protocols. The cDNA pellet for DMS/SHAPE-LMPCR was redissolved in RNase-free water and additions were made resulting in final concentrations of 70 μM of DNA linker with a 5′-phosphate and a 3′-3-Carbon spacer group (5′p, 3′C3), 50 mM MOPS (pH 7.5), 10 mM KCl, 5 mM MgCl 2 , 1 mM DTT, 0.05 mM ATP, 2.5 mM MnCl 2 and 200 U total Circligase I in a 20 μl reaction. The ligation was performed at 65 °C for 12 h, followed by heating at 85 °C for 15 min to deactivate the Circligase I. The solution was then phenol chloroform extracted, applied to an illustra MicroSpin S-200 HR column (GE Healthcare Life Sciences) following the manufacturer’s protocol and then the ligated cDNA in the filtrate was subjected to ethanol precipitation. Selective PCR amplification The ligated cDNA samples were dissolved in 10 μl of water and 1 μl of the reaction was used for the PCR reaction. The PCR reaction contained final concentrations of 0.5 μM forward primer, 0.5 μM of gene-specific reverse primer, 1 μl of ~500,000 cpm μl −1 32 P-labelled gene-specific reverse primer (omitted for CE detection), 200 μM dNTPs, 1X ThermoPol reaction buffer and 1.25U of NEB Taq DNA polymerase in 25 μl. For CE, 0.5 μM of 6-FAM (fluorescein)-labeled gene-specific reverse primer was used instead. The PCR protocol consisted of 1 cycle of 95 °C for 3 min; 25–35 cycles of 95 °C for 1 min, 60 °C for 45 s and 72 °C for 1 min; followed by 72 °C for 10 min and then cooling to 4 °C. For PAGE, the reaction mixture was mixed with an equal volume of 2X stop solution, which contained 100% deionized formamide, 20 mM Tris (pH 7.5), 40 mM EDTA and xylene cyanol and bromophenol blue dye for tracking, while for CE, 1 μl of the products was mixed with 0.5 μl of LIZ-500 size standard (ABI Cat. 602912) and 10 μl of deionized formamide (Applied Biosystems). Data collection For PAGE-based DMS/SHAPE-RT and DMS/SHAPE-LMPCR, products were size fractionated on 8.3 M urea-8% polyacrylamide gels for DNA size separation. To help denature the DNA, the temperature of the glass plates was maintained at ~55–60 °C, which was achieved by a power of 90–100 W. Gels were dried under vacuum and heat. Gel images were collected with a Typhoon PhosphorImager 9410, and bands were quantified using SAFA [38] or ImageQuant 5.2. For CE-based SHAPE-LMPCR, products were size fractionated on a 50 cm capillary array with POP7 matrix using a 3730XL DNA Analyzer (Applied Biosystems, Foster City, CA). The run module was set to the following parameters: voltage 15 kV, T =66 °C, injection time=10 s. Product sizes were assessed using Peak Scanner v1.0 software (Applied Biosystems, Foster City, CA). Data processing and analysis The DMS or SHAPE data were processed according to the literature [7] , [8] . In summary, the differences in band intensity between (+)DMS and (−)DMS or (+)SHAPE and (−)SHAPE reactions were calculated. The nucleotide identity of each band was identified from dideoxy sequencing lanes or the DNA size marker lane. Since DMS specifically targets the Watson–Crick position of A and C nucleotides, the G and U nucleotides were not included during signal processing. Normalized DMS or SHAPE reactivity was generated based on the 2/8% rule [7] , [8] . Using DMS as an example, the top 2% of the most reactive A and C nucleotide intensities were designated as outliers and removed from the pool for averaging. The next 8% of most reactive A and C nucleotide intensities were averaged, and all A and C nucleotide intensities, including the outliers, were divided by this average value to obtain normalized DMS reactivity. The same procedure was followed for SHAPE, except that all four nucleotides were used for the normalization. The normalized DMS/SHAPE reactivities were then plotted for further analysis. (See Figs 3 and 7 and Supplementary Fig. S4 ). Statistical analyses For comparison of in vitro and in vivo DMS/SHAPE reactivites, Pearson correlation tests were performed. The Pearson’s correlation coefficient is a statistical measure of the linear correlation between two variables, which yields a value ranging from −1 (perfect negative correlation) to 1 (perfect positive correlation), where zero indicates no correlation. RNA structure determination In vitro and in vivo DMS/SHAPE-constrained RNA structure determination was performed at the RNA Mapping Data Bank (RMDB) structure server website [39] ( http://rmdb.stanford.edu/structureserver/ ). Briefly, the normalized and quantified DMS/SHAPE reactivities were formatted and input into the website as pseudo-energy constraints along with the RNA sequence. Subsequently, the RNA was folded at 25 °C using default slope and intercept parameters. This server uses RNAstructure [40] , [41] ( http://rna.urmc.rochester.edu/index.html ) as the backend. Multiple sequence alignment and RNA structure prediction U12 snRNA sequences were obtained from Phytozome v9.1 (ref. 42 ) ( http://www.phytozome.net/ ) or NCBI GenBank (ref. 43 ) ( http://www.ncbi.nlm.nih.gov/genbank/ ). The plant U12 snRNA sequences were aligned using Clustal W2 [44] ( http://www.ebi.ac.uk/Tools/msa/clustalw2/ ). The sequences were submitted to TurboFold [45] ( http://rna.urmc.rochester.edu/RNAstructureWeb/Servers/TurboFold/TurboFold.html ) to derive a secondary structure of U12 snRNA for A. thaliana , based on consensus among the designated sequences. Expression analysis by quantitative RT-PCR Total RNA was extracted from 5-day-old A. thaliana etiolated seedlings using the RNeasy Plant Mini Kit (Qiagen) according to the manufacturer’s protocol. RNA was quantified spectrophotometrically (Nanodrop-2000; NanoDrop Technologies) and RNA quality was checked by gel electrophoresis to confirm that rRNA bands were intact. The total RNA was treated with TURBO DNase (Ambion) according to the manufacturer’s instructions and subsequently phenol chloroform extracted and ethanol precipitated. The total RNA was dissolved in RNase-free water and stored at −20 °C before use. Total cDNA was prepared from 500 ng of total RNA with the SuperScript III first-strand synthesis system for RT-PCR (Life Technologies, Invitrogen) using random hexamers and following the manufacturer’s instructions. Next, qRT–PCR was performed using a premix containing SYBR-Green intercalating dye (Bio-Rad) and selected gene-specific primer sets. The positions of the oligonucleotide primers for each RNA of interest used for qRT–PCR were chosen such that the size of all PCR products was between 100 and 150 bp. The suitability of the oligonucleotide sequences in terms of efficiency of annealing was evaluated in advance using the mFold [46] and Primer 3 programs [47] . Primer efficiency tests were performed on each of the four qRT-PCR primer sets. The efficiencies of all primer sets were found to be highly similar to each other and within the acceptable range. Primers for each gene are provided in Supplementary Table S2 . Threshold cycle ( C t ) values in qRT-PCR experiments were averaged across three technical replicates. Three independent biological replicates were performed. The averaged C t value of the three biological replicates was used for the calculation of relative expression, and the s.d. was generated from the three biological replicates. The data obtained were analysed with IQ5 software (Bio-Rad). How to cite this article: Kwok, C. K. et al . Determination of in vivo RNA structure in low-abundance transcripts. Nat. Commun. 4:2971 doi: 10.1038/ncomms3971 (2013).